Stepwise self-assembly of C60mediated by atomic scale moiré magnifiers Self-assembly of atoms or molecules on a crystal surface is considered one of the most promising methods to create molecular devices. Here we report a stepwise self-assembly of C 60 molecules into islands with unusual shapes and preferred sizes on a gold–indium-covered Si(111) surface. Specifically, 19-mer islands prefer a non-compact boomerang shape, whereas hexagonal 37-mer islands exhibit extraordinarily enhanced stability and abundance. The stepwise self-assembly is mediated by the moiré interference between an island with its underlying lattice, which essentially maps out the adsorption-energy landscape of a C 60 on different positions of the surface with a lateral magnification factor and dictates the probability for the subsequent attachment of C 60 to an island’s periphery. Our discovery suggests a new method for exploiting the moiré interference to dynamically assist the self-assembly of particles and provides an unexplored tactic of engineering atomic scale moiré magnifiers to facilitate the growth of monodispersed mesoscopic structures. Self-assembly of atoms or molecules on a crystal surface is a potential route to creating molecular devices [1] . Researchers have been exploiting the interaction between a particle and a surface to help particles self-assemble into increasingly larger structures with specific shape and size that determine their physical properties. To create structures larger than a typical crystal unit cell, surfaces with large superstructures of quasi-periodic inhomogeneous adsorption sites, for example, Au(111)22 × √3 ‘herringbone’ reconstruction [2] , [3] , vicinal Au(11 12 12) (refs 4 , 5 ) surfaces and the strain-relief patterns formed by Ag on Pt(111) (refs 6 , 7 ), have been exploited as ‘anchor sites’ to assist the aggregation of particles. In such template-guided particle assembly, the surface provides a quasi-periodic array of static potential wells with a large lateral size for the particles to nucleate and aggregate into an ensemble of islands. One simply hopes that the potential wells are deep enough for the particles to be evenly distributed into every well to reduce the island size dispersion. Unfortunately, these attempts have had limited success because the wells usually have insufficiently depth or dissimilar lateral geometry. It is therefore important to search for new schemes of particle-surface interaction that could guide the self-assembly of particles with an effect beyond those provided by static strain-relief patterns and facilitate the fabrication of complex supramolecular structures, paving ways towards future molecular devices. Here we report the discovery of a new scheme of particle self-assembly mediated by moiré interference between an already assembled island and its underlying surface lattice. The system studied was the self-assembly of C 60 molecules on an gold–indium (Au–In)-covered Si(111) surfaces. Using C 60 as a prototype molecule for studying particle assembly is attractive because of its compact and highly symmetric structure, and the interaction between two C 60 molecules is well characterized. Furthermore, C 60 has the ability to accept electrons from other molecules, atoms and surfaces [2] , therefore an ensemble of monodispersed C 60 clusters has the potential to exhibit interesting electronic properties, which could be the foundation for its applications in nanodevices. On the other hand, the Au–In-covered Si(111) surface is a highly homogeneous surface at room temperature (RT) [8] , [9] . In previous studies, when an overlayer of C 60 molecules adsorb on such homogenous Si(111)√3 × √3-(Au,In) surface, two phase of hexagonal close-packed C 60 lattice with different lattice orientations have been observed [10] . One phase, referred as A-phase, show moiré pattern with periodical bright spots in scanning tunnelling microscope (STM) images, and the other, referred as B-phase, show smooth appearance in STM images. As described later, the moiré interference of A-phase has important roles for C 60 self-assembly. In contrast to the typically observed continuous aggregation of particles, C 60 molecules on Au–In-covered Si(111) show stepwise self-assembly, forming islands with unusual shapes and preferred sizes. Specifically, 19-mer islands prefer a non-compact boomerang shape, whereas hexagonal 37-mer islands with 2,220 carbon atoms exhibit extraordinarily enhanced stability and abundance. The stepwise self-assembly is found to be mediated by the moiré interference between an already self-assembled island with its underlying lattice, which essentially maps out the adsorption-energy landscape of a C 60 on different lateral sites of the surface with a lateral magnification factor. This atomic scale ‘moiré magnifier’ dictates the probability for a C 60 to attach subsequently to a site along the peripheral of an existing island. Every step in the self-assembly corresponds to a dramatic drop in an island’s growth rate when it reaches certain shape and size determined by the moiré interference pattern. Our discovery points to a new method for exploiting the moiré interference between an existing structure with the underlying surface to dynamically assist the subsequent self-assembly of particles and provides an unexplored tactic of engineering atomic scale moiré magnifier [11] to facilitate the growth of monodispersed mesoscopic structures with atomic precision. C 60 islands with unusual shapes and magic sizes The preparation and properties of the Si(111)√3 × √3-(Au, In) surface are described in Methods. In brief, In adsorption onto the Si(111)-√3 × √3-Au surface at RT followed by annealing produces a highly homogeneous surface, which preserves its original conjugate honeycomb trimer atomic arrangement [12] , [13] . The ~0.15 monolayer (ML) of In on the surface forms a two-dimensional (2D) gas of mobile adatoms that solidifies at ~100 K. The C 60 deposited onto the Si(111)√3 × √3-(Au,In) surface at 110 K self-assemble into 2D clusters and islands of different sizes and irregular shapes as shown in Supplementary Fig. S1a . After short RT annealing, the clusters and islands grow while their shapes change from irregular to crystalline-like with a 2D hexagonal closed packing (HCP), as shown in Fig. 1a . Their crystal orientations point to either 0 or 19.1° with respect to the main crystallographic direction of the underlying Si(111) surface, as indicated by phase A and B, respectively. The most striking feature in the images is the presence of considerable number of islands with unusual shapes like boomerang (19-mer), zigzag (30-mer) and stadium (13-mer), as shown in the insets of Fig. 1a . As these islands are not compact, that is, without geometric shell closure, and they are unexpected based on energetic arguments, their presence immediately raises an interesting question: what drives them to assume such unusual shapes? 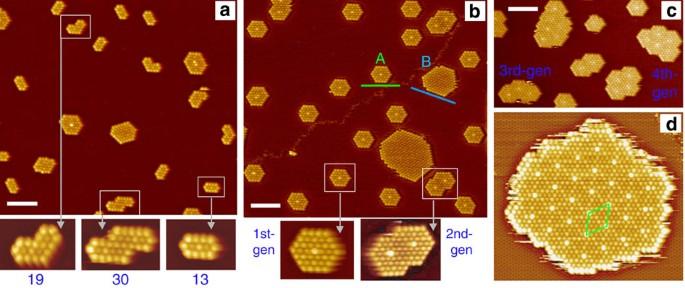Figure 1:C60islands with unusual shapes and magic sizes. (a) Immediately after warming up a sample (0.1 ML of C60) prepared at 115 K to RT, small (10–30 of C60) ordered islands with non-compact shapes such as boomerang (19-mer), zigzag (30-mer) and stadium (13-mer) are formed. (b) After annealing the sample (0.2 ML of C60) at RT for 2 h, medium-size islands with compact shapes appear. Most islands have the shape of a hexagon or two overlapped hexagons, each possessing a characteristic central bright spot, which is used as an indicator of an island’s generation. The green and blue lines show lattice orientations of the A- and B-phase islands, respectively. (c) Deposition of higher coverage of C60at RT leads to the formation of larger islands with characteristic shape of overlapped hexagons. (d) A large island formed by deposition of C60at RT exhibits moiré interference pattern with similar characteristic periodical bright spots. The green rhombus indicates the unit cell of the moiré pattern. Scale bar, 10 nm (a–c). Figure 1: C 60 islands with unusual shapes and magic sizes. ( a ) Immediately after warming up a sample (0.1 ML of C 60 ) prepared at 115 K to RT, small (10–30 of C 60 ) ordered islands with non-compact shapes such as boomerang (19-mer), zigzag (30-mer) and stadium (13-mer) are formed. ( b ) After annealing the sample (0.2 ML of C 60 ) at RT for 2 h, medium-size islands with compact shapes appear. Most islands have the shape of a hexagon or two overlapped hexagons, each possessing a characteristic central bright spot, which is used as an indicator of an island’s generation. The green and blue lines show lattice orientations of the A- and B-phase islands, respectively. ( c ) Deposition of higher coverage of C 60 at RT leads to the formation of larger islands with characteristic shape of overlapped hexagons. ( d ) A large island formed by deposition of C 60 at RT exhibits moiré interference pattern with similar characteristic periodical bright spots. The green rhombus indicates the unit cell of the moiré pattern. Scale bar, 10 nm ( a – c ). Full size image Prolonged RT annealing leads to further ripening of C 60 clusters and the formation of larger islands with characteristic shapes of isolated hexagon or overlapped hexagons ( Fig. 1b ), which all have distinct bright spots in their centres (insects). The spots appear brighter in both the empty- and filled-sate STM images, indicating that the central C 60 is likely to be geometrically higher (0.1–0.2 nm) than its neighbours. The islands have two bands of preferred sizes at 37–44 and 70–80 while the as-deposited clusters have a broad continuously decaying size distribution with a mean value of ~15, as shown in Supplementary Fig. S1b . Again, these observations raise an interesting question: what is the thermodynamic driving force for the preference in the islands’ size and the characteristic shape of overlapped hexagons with distinct central bright spots? Samples with higher coverage of C 60 form larger islands with the same characteristic shape of overlapped hexagons and distinct central bright spots ( Fig. 1c ) after RT annealing. Samples prepared by depositing C 60 at RT leads to the formation of even larger islands with a periodical pattern of similar bright spots, as shown by the example in Fig. 1d . Such a pattern is reminiscent of the moiré interference pattern commonly observed when two grids are overlaid at an angle, or when they have slightly different mesh sizes. By comparing the apparent heights and separation of the bright spots in Fig. 1d with those in Fig. 1b , it is evident that all the bright spots originated from the same moiré interference between the HCP lattice of a C 60 island and the underlying surface lattice. Therefore, the distinct bright spots in the centre of every hexagon on an island can be taken as a trait for identifying this particular species that eventually grow into large islands with the characteristic moiré pattern of periodical bright spots. For this reason, we shall refer to such A-phase islands with zero, one and two bright spots as zero-, first and second-generation islands, respectively, and so on so forth. We note that A-phase islands dominate the island populations at RT while they are taken over by B-phase islands when temperature is increased to 380 K. An ensemble of monodispersed C 60 islands In situ STM observations of C 60 islands ( Supplementary Movie 1 ) during RT annealing reveal continuous changes in their sizes and shapes via active exchange of mobile C 60 on the surface. An example of particular interest shows how a 48-mer firstly becomes a 44-mer and eventually a 37-mer, as shown in Fig. 2a–c . Note that the nearby 37-mer preserves its size and shape during the same course. This result indicates that the 37-mer is more stable than the 44-mer and 48-mer, although both of which have geometric shell closure. As demonstrated by the histogram in Fig. 2d , after a short annealing time (30 min), the population consists primarily of 48-mers and secondarily of 44-mers and 52-mers. After 24 h of annealing, 37-mers become dominant, whereas a small number of 44-mers survive. After 48 h, the system become essentially monodispersed with the 37-mers constituting about 80% of the islands, as demonstrated clearly in Fig. 2d . Because a 37-mer consists of exactly 2,220 carbon atoms, this system constitutes an ensemble of monodispersed mesoscopic structure with an unprecedented large size while maintaining their atomic precision. 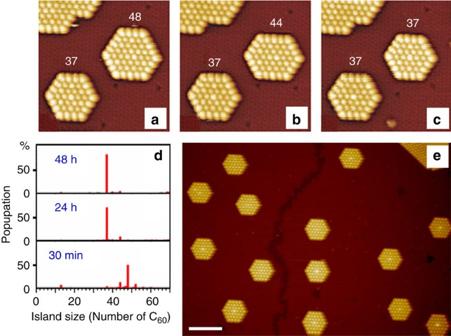Figure 2: Enhanced stability of hexagonal 37-mers. (a–c) A sequence of STM images showing the evolution of an island from 48-mer to 44-mer and finally to 37-mer during RT annealing. (d) Island size distributions after various annealing time. Short (30 min) annealing leads to an overshoot of the island sizes above the final size of 37. Long-time annealing reduces island sizes and finally tunes 80% of the islands to most preferred size of 37. (e) Images showing exclusive selections of 37-mers after RT annealing for 48 h. Scale bar, 10 nm. Figure 2: Enhanced stability of hexagonal 37-mers. ( a – c ) A sequence of STM images showing the evolution of an island from 48-mer to 44-mer and finally to 37-mer during RT annealing. ( d ) Island size distributions after various annealing time. Short (30 min) annealing leads to an overshoot of the island sizes above the final size of 37. Long-time annealing reduces island sizes and finally tunes 80% of the islands to most preferred size of 37. ( e ) Images showing exclusive selections of 37-mers after RT annealing for 48 h. Scale bar, 10 nm. Full size image Before achieving exclusive selection of the 37-mers, the evolution in the island size distribution exhibited an unusual ‘overshoot’ in the island growth process. Typical system of island growth proceeds with monotonic increase in the maximum of the size distribution while this system starts with a maximum at 44 and then ‘grow’ to a smaller value of 37. Such unusual growth behaviour indicates that an island’s Gibbs energy as a function of its size has a broad minimum centred at 37 and extending all the way to at least 52. Depending on the coverage of C 60 and the initial condition of deposition, as well as the thermal history of the system, the maximum of the size distribution could be initially larger than the most favoured size corresponding to the minimum in the Gibbs energy. The thermodynamic driving force eventually attracts most islands back to become the most favoured 37-mer through exchange of C 60 along the peripherals of the islands. In other words, the size distribution is influenced by the ‘molecular vapour’ around the islands. During deposition, the ‘vapour pressure’ around the island is high. At RT, even without the deposition flux, there are still mobile molecules on the surface. Given enough time, the number of these diffusing molecules will decrease because molecules are captured by some very large islands for example. At this stage, the ‘oversized’ islands, 48 or 44 for instance will get rid of some molecules by a process similar to sublimation. The extraordinary stability of the 37-mer in comparison with other first-generation C 60 islands with geometric shell closure such as the 44-mer and 48-mer appears to hold the key to understanding the preference in islands’ sizes and shapes. To better characterize the structure of a 37-mer, we use its surrounding Si(111)√3 × √3-(Au, In) lattice to measure the lateral positions of its constituent C 60 s, as illustrated in Supplementary Fig. S2a . Based on the detailed measurement, we conclude that the lateral position of its central bright spot is directly on top of an Au trimer on the underlying lattice. Because the C 60 s on the Au trimers appear as bright spots in both empty (+2 and +1 V) and filled (−2 and −1 V) state images [10] , and ~1/30 of the bright C 60 in 37-mers and other islands of different generations are missing (see Supplementary Fig. S2b ), it is most likely that the bright C 60 s are geometrically higher and it is also energetically unfavourable for a C 60 to sit on top of a Au trimer. Stepwise self-assembly of a C 60 island The enhanced stability of higher-generation islands of certain sizes and shapes is further demonstrated by in situ STM monitoring of the self-assembly of C 60 during RT deposition ( Supplementary Movie 2 ). 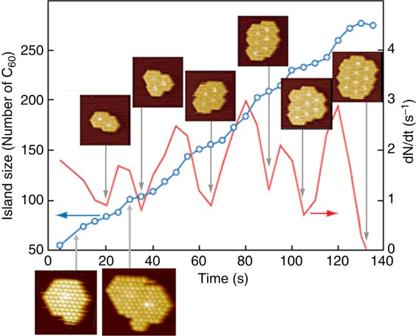Figure 3:Stepwise self-assembly of a C60island. The blue curve shows the island size as a function of C60deposition time and the red curve is the derivative of blue curve, that is, growth rate. The blue curve show many flat sections, during which the island exhibits the shape of overlapped hexagons and its growth rate reaches a local minimum, as demonstrated by the upper insets for second- to tenth-generation islands. The lower insets show two intermediate islands exhibiting characteristic budding from their corners as they grow from one generation to the next. Figure 3 shows the size of an island as a function of deposition time. When it grows from the second generation to the tenth generation, its growth rate, as shown by the derivative of the island size (red line) in Fig. 3 , drops to a local minimum from time to time. Such a stepwise growth is qualitatively very different from a typical continuous growth of an island formed by random aggregation of surrounding particles. (We note that a reverse process of stepwise decay of Ag adatom islands has been observed on Ag(111) surfaces [14] ) The growth rate reaches a local minimum whenever the island assumes a shape covering certain number of overlapped hexagons with central bright spots, as shown by the upper insets in Fig. 3 . To draw an analogy to the well-known geometric and electronic shell closure [15] that lead to the preference in certain cluster sizes, we will refer to the phenomenon as ‘moiré shell closure’ that leads to the dramatical reduction in the growth rate at certain preferred island size. Figure 3: Stepwise self-assembly of a C 60 island. The blue curve shows the island size as a function of C 60 deposition time and the red curve is the derivative of blue curve, that is, growth rate. The blue curve show many flat sections, during which the island exhibits the shape of overlapped hexagons and its growth rate reaches a local minimum, as demonstrated by the upper insets for second- to tenth-generation islands. The lower insets show two intermediate islands exhibiting characteristic budding from their corners as they grow from one generation to the next. Full size image It is surprising to note that dN/dt for the 8th- and 10th-generation island is lower than that for the smaller islands because larger islands are expected to be able to capture more molecules in unit time. This systematic decline in the growth rate of this A-phase island as it grew beyond the 6th generation is counterintuitive even if one considers the size-dependent stability and the statistical fluctuation. We believe the decline was caused by the presence of a much larger B-phase island to its left, as shown in Supplementary Fig. S3a . As B-phase are more stable thermodynamically, such a nearby B-phase island would act as a sink to create a ‘low vapour pressure’ zone between the two islands, which is supported by the fact that the growth front never appeared on left side of the A-phase island since the beginning of the growth ( Supplementary Fig. S3b ). The competition between the two islands for C 60 molecules became the dominant effect at the latter stage of the growth such that the Otswald-ripening-like process favoured the growth of the larger B-phase island, whereas reducing the growth rate of the A-phase island. (see Supplementary Note 1 ). To better understand this new type of shell closure, it is helpful to look for any trend in the ‘cracking’ of its shell as an island grows from one generation to the next. The two lower insets of Fig. 3 depict the detailed view of the interesting characteristic of ‘budding’ from the corners of the first- and second-generation islands. It suggests that the regions near the corners of an island with moiré shell closure are the lower-energy regions in the adsorption-energy landscape and favoured by the mobile C 60 s in the surrounding. The details of such moiré shell closure and its implications to the stepwise growth of higher generation of islands with different local geometry are described in Supplementary Note 1 and Supplementary Fig. S3b . Theoretical calculations are evoked to help unravel the mystery of the stepwise self-assembly and its correlation to the moiré-interference pattern. The first step is to calculate the adsorption energy of a C 60 on different lateral sites of the Si(111)√3 × √3-(Au, In) surface, using the Vienna ab initio Simulation Package based on density functional theory with projector-augmented wave pseudopotentials. Because van der Waals forces are important in C 60 –metal and C 60 –C 60 interactions [16] , we use non-local van der Waals exchange-correlation function (vdW-DF2) [17] , [18] , [19] to obtain more accurate binding energies (see Supplementary Note 2 and Supplementary Figs S4–S7 ). The calculated adsorption energy of a C 60 as a function of its lateral position, which will be referred simply as C 60 adsorption-energy landscape hereafter, is shown as a 3D surface plot in Fig. 4a . The landscape exhibits only one peak located on top of the Au trimer. 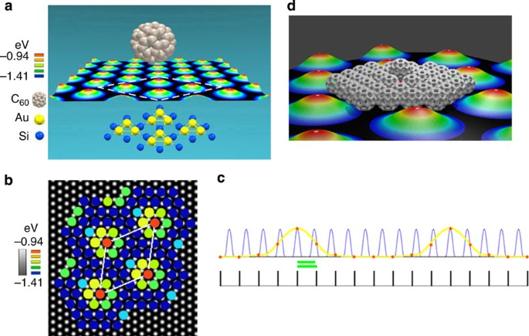Figure 4:Calculated adsorption energy of an individual C60and C60s in an island. (a) 3D representation of the adsorption energy of an individual C60as a function of its lateral position on the surface derived fromab initiocalculation. An atomic model of an area indicated by the white rhombus (mobile In is neglected) is shown. The energy reaches the maximum on the centre of a Au trimer. (b) Simulated adsorption energy of C60s in a fourth-generation island with minimized total energy. The energy is represented by different colour. The rhombus indicates a unit cell of the moiré pattern. (c) Schematics demonstrating the lateral magnifying effect when a wave is sampled discretely by another wave with slightly different period. (d) 3D representation of the C60s in a 37-mer and the MPF. Every edge of the island is confined by a potential peak, and the central C60occupies the apex of a peak, closely resembling the characteristic bright spot observed on the STM image (the apparent height of the central C60is not drawn to scale). Figure 4: Calculated adsorption energy of an individual C 60 and C 60 s in an island. ( a ) 3D representation of the adsorption energy of an individual C 60 as a function of its lateral position on the surface derived from ab initio calculation. An atomic model of an area indicated by the white rhombus (mobile In is neglected) is shown. The energy reaches the maximum on the centre of a Au trimer. ( b ) Simulated adsorption energy of C 60 s in a fourth-generation island with minimized total energy. The energy is represented by different colour. The rhombus indicates a unit cell of the moiré pattern. ( c ) Schematics demonstrating the lateral magnifying effect when a wave is sampled discretely by another wave with slightly different period. ( d ) 3D representation of the C 60 s in a 37-mer and the MPF. Every edge of the island is confined by a potential peak, and the central C 60 occupies the apex of a peak, closely resembling the characteristic bright spot observed on the STM image (the apparent height of the central C 60 is not drawn to scale). Full size image Next is to calculate the total adsorption energy of an island based on the adsorption-energy landscape of an individual C 60 derived from ab initio calculation ( Fig. 4a ). In this classical calculation (see Supplementary Note 2 and Supplementary Figs S8 and S9 ), an island is simulated by a group of C 60 s arranged with a fixed HCP geometry in which every C 60 has its adsorption energy determined by its lateral position inside a √3 × √3 unit cell of the underlying surface. Because the sizes of a C 60 and the √3 × √3 unit cell are both ~1 nm, each cell can only accommodate one C 60 . The array of adsorption energy for every C 60 on an island is equivalent to a discrete map that samples different points of the adsorption-energy landscape. Therefore, the total adsorption energy of an island is simply the sum of these sampled values. To find the most stable location and orientation of an island, which is treated as a rigid body, we just need to scan its centre-of-mass across a unit cell and its orientation through 360° to find the minimum energy. We note that our simulation is a simplified version of the Frenkel–Kontorova model commonly used to describe the dislocation lines and moiré patterns in the growth of metal films on metal surfaces such as Cu on Ru(0001) [20] , [21] . As an example of the simulation, Fig. 4b shows the most stable orientation and location for a fourth-generation island. Palettes of different colours are used to represent C 60 with different adsorption energy. The island’s lattice orientation aligns with the main crystallographic direction of the underlying Si(111), consistent with the experiment. The island has four high adsorption-energy peaks resembling the four bright spots on a unit cell of the moiré pattern. The profiles connecting the adsorption energy of the C 60 on the island appear to be similar to that of the adsorption-energy landscape for an individual C 60 on the Si(111)√3 × √3-(Au, In) lattice ( Fig. 4a ), except its lateral scale has been magnified. To help illustrate such a magnifying mapping of the adsorption-energy landscape, Fig. 4c shows a 1D analogy to the present case, in which the periods of the potential energy and the discrete mapping function are slightly different. The small difference leads to the sequential sampling of different points of the potential energy surface. The collection of the sampled points constitutes a potential function and equals to the original adsorption-energy landscape magnified laterally by a factor inversely proportional to the small difference. Such moiré-magnifier effect [11] , which is well known in many branches of physics such as optics, sound and radio wave transmission, is essentially the result of the ‘beating’ between the lattice of the C 60 island and that of the underlying surface. In other words, the ‘beating’, or interference, creates the long wavelength √19 × √19 superlattice of moiré pattern, which has a negligible lattice mismatch of only ~0.15% with respect to the period of the structure along certain orientation of surface lattice. For simplicity, we will refer to the laterally magnified discrete mapping of the C 60 adsorption-energy landscape as the moiré potential field (MPF) hereafter. Figure 4d shows a three-dimensional (3D) representation of a 37-mer superimposed on the MPF, clearly indicating that its edges are confined by potential peaks and its central C 60 occupies the summit of a peak. The apparent ‘moiré shell closure’ imposed by the surrounding peaks could account for its extraordinarily enhanced stability and therefore the excellent monodispersity in the island size distribution. To be noted, the validity of the MPF depends on the HCP of the C 60 in an island. To maintain the HCP geometry, the binding energy between two neighbouring C 60 ( Supplementary Figs S6 and S7 ) must significantly exceed the gradient of the MPF. Or else, cracks could form on an island, rendering the MPF invalid. It appears that the layer of HCP C 60 s in this particular system could be treated like a membrane that deforms locally to accommodate the local variation in the MPF. To help visualise how the moiré interference dynamically assists the self-organization of C 60 into islands with unusual shapes and preferred sizes, we superimpose some particular islands on a large island with moiré patterns ( Fig. 5a ) and plot the MPF surrounding these islands ( Fig. 5b ). As shown in Fig. 5a , 7-mer, 13-mer and 19-mer can be arranged in such ways that they are surrounded by bright spots, providing experimental evidence that the formation of such islands are governed by a simple rule to avoid the creation of bright spots, that is, all the C 60 s in the island avoid occupying the sites on top of the Au trimers. For comparisons, the MPF surrounding these islands are illustrated in Fig. 5b . For the 7-mer, only the most compact hexagonal isomer survives because its size is small enough to fit into the potential gorge of the field. The 13-mer is elongated horizontally because its vertical dimension is restricted by two potential peaks. The 19-mer has to bend into the unusual boomerang shape to go around a peak and fit into the gorge surrounding the peaks. The same mechanism leads to the bending and formation of the 30-mer ‘zigzag’ island (not shown). Annealing at RT forces the 48-mer and 44-mer with geometric shell closure to give up some of their peripheral C 60 s with higher potential energies and become the most stable regular hexagonal 37-mer with both geometric and moiré shell closure. The 67-mer illustrates the ‘budding’ from a corner of a first-generation island as it begins to grow into a second-generation island, similar to the first lower inset of Fig. 3 . The MPF clear indicates that the regions near the corners have lower potential energy for the attachment of C 60 . Once a corner region is occupied, the island can grow around a peak. Gradually, C 60 s pile up on the slope and eventually reach the summit, forming a next-generation island with an additional bright spot. For a peak much higher than the present case, an island would grow around the peak, forming a network of connected ring-shape structure (see Supplementary Fig. S10c ). On the other hand, if the MPFs were made of an array of wells, the shapes of islands would be compact, similar to the geometric shell closure (see Supplementary Fig. S10b ). 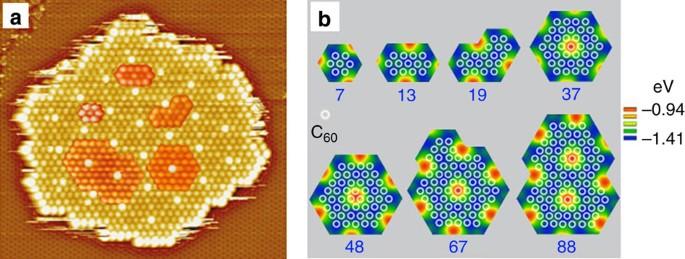Figure 5:C60islands superimposed on aMPF. (a) Magic islands are superimposed on a large island with moiré patterns. 7-mer, 13-mer and 19-mer can be arranged such that their borders avoid the bright spots. (b) The peaks of the MPF block the growth of islands and lead to the preference in the shape and size of islands, as well as an unique ‘budding’ from the corners of an island with ‘moiré-shell closure’. Figure 5: C 60 islands superimposed on a MPF. ( a ) Magic islands are superimposed on a large island with moiré patterns. 7-mer, 13-mer and 19-mer can be arranged such that their borders avoid the bright spots. ( b ) The peaks of the MPF block the growth of islands and lead to the preference in the shape and size of islands, as well as an unique ‘budding’ from the corners of an island with ‘moiré-shell closure’. Full size image To be emphasized, the MPF shown in Fig. 5b should be discrete but appears continuous for better visualization. It can only be used for describing the adsorption energy of a C 60 that is already part of the island or yet to be added to the peripheral of the island following the same HCP geometry of the existing island. In other words, the continuous potential field in Fig. 5b does not exist in real space, however, it is a very useful conceptual tool to help predict the probability for a C 60 to attach to different sites along the peripheral of an existing C 60 island and reveal the origins of islands’ size/shape preferences in C 60 islands. We then discuss the effects of In, which has key roles in the formation of moiré pattern of A-phase overlayers and the stepwise self-assembly of C 60 islands. According to STM images [8] and angle-resolved photoelectron spectroscopy measurments [9] taken at RT, ~0.15 ML of In mobile adatoms on the Si(111) √3 × √3-(Au, In) surface results in the formation of 2D electron gas, which is distributed as honeycomb network excluding the sites on top of the Au trimers. Because the distributions of free electron gas exclude Au-trimer sites, we would expect less charge transfer from surfaces to the C 60 s on Au-trimer sites, as supported by our STS observations ( Supplementary Fig. S11 ) that lowest unoccupied molecular orbital states of C 60 molecules on the bright regions (that is, on Au-trimer sites) are higher than that on the dark regions. Therefore, C 60 s on Au-trimer sites have weaker adsorption energy, as supported by the missing C 60 in central bright region of 37-mer ( Supplementary Fig. S2b ), and are geometrically higher, showing bright spots in empty and filled state STM images [10] . These observations suggest that at RT the In atoms provide delocalized electrons to the honeycomb network excluding the Au-trimer sites, which is also supported by the results of our theoretical calculations. When temperature is cooled to 110 K, In atoms and the 2D electron gas are frozen and no longer distributed evenly on honeycomb network ( Supplementary Fig. S1a ), which coincides with the disappearance of ~1/4 of the bright spots from the large A-phase islands [10] . We therefore speculate that, at low temperature, the local variation of the In atoms could affect the local electron density near the C 60 in the centre of a honeycomb and its brightness. The effect of the moiré magnifier facilitates the creation of monodispersed structures with lateral sizes much larger than a typical crystal unit cell. It could be exploited as a new type of substrate-assisted particle self-assembly for the construction and size selection of large molecular devices. Such a new approach to the substrate-assisted self-assembly of size-selected structures via ‘moiré shell closure’ is conceptually very different from the previous approach that uses surfaces with large superstructures of quasi-periodic inhomogeneous adsorption sites [2] , [3] , [4] , [5] , [6] , [7] as ‘anchor sites’ to assist the aggregation of particles and achieves size selection. The creation of an ensemble of monodispersed surface-clusters of 37-mer is a remarkable achievement, especially, in light of fact that the largest monodispersed surface-clusters that has been reported to date contains merely 10 galliums [22] . This dramatic increase in the cluster size is primarily due to the use of C 60 as building blocks rather than atoms. For this tactic to work, one intuitively would expect the need of a potential field with a larger periodicity to accommodate the molecule. An atomic scale moiré magnifier is an unexpected alternative to substrate-assisted self-assembly of particles into ordered structures, providing a new tactic to growing larger monodispersed mesoscopic structures with atomic precision. Preparations of C 60 islands on In–Au-covered Si(111) Our experiments were performed with an Omicron STM operating in an ultrahigh vacuum (2.0 × 10 −10 Torr). Atomically clean Si(111)-7 × 7 surfaces were prepared in situ by flashing to 1280 °C after the samples were first outgassed at 600 °C for several hours. Gold was deposited from an Au-wrapped tungsten filament, indium from Ta crucible and C 60 fullerenes from a resistively heated Mo crucible. For sample preparations, first, deposition of 1 ML of Au on Si(111) surfaces at 700 °C leads to the formation of Si(111)√3 × √3-Au surfaces. The surface shows up in STM image as combination of dark regions corresponding to domains of commensurate √3 × √3-Au phase and a network of bright lines corresponding to domain walls. Second, 0.5 ML of In is deposited onto the Si(111)√3 × √3-Au at RT followed by brief annealing at 600 °C, which results in complete elimination of the domain walls but preserving the original Si(111)√3 × √3-Au conjugate conjugate honeycomb trimer structure. We note that only ~0.15 ML of In is left at the resultant homogeneous surface. The In adatoms form a 2D gas of mobile atoms at RT, producing a characteristic honeycomb pattern in the STM images, and can be frozen upon cooling the sample to ~100K ( Supplementary Fig. S1 ). Deposition of C 60 onto In–Au-covered Si(111) surfaces at RT results in the formation of hexagonal close-packed C 60 islands with two different lattice orientations. The lattice vectors of A-phase islands with bright spots are aligned along the main crystallographic direction of the underlying Si(111) and those of B-phase islands are rotated by 19.1°. In situ monitoring of C 60 island growth In our in situ monitoring of island growth, each dosing step included two stages: turn on the C 60 flux for 5 s and then turn off the flux for 5 s. The images were taken at the end of the second stage. The data acquisition time for an image was ~25 s. How to cite this article: Gruznev, D. V. et al . Stepwise self-assembly of C 60 mediated by atomic scale moiré magnifiers. Nat. Commun. 4:1679 doi: 10.1038/ncomms2706 (2013).